Room-temperature-concerted switch made of a binary atom cluster Single-atom/molecule manipulation for fabricating an atomic-scale switching device is a promising technology for nanoelectronics. So far, scanning probe microscopy studies have demonstrated several atomic-scale switches, mostly in cryogenic environments. Although a high-performance switch at room temperature is essential for practical applications, this remains a challenging obstacle to overcome. Here we report a room-temperature switch composed of a binary atom cluster on the semiconductor surface. Distinctly different types of manipulation techniques enable the construction of an atomically defined binary cluster and the electronic switching of the conformations, either unidirectionally or bidirectionally. The switching process involves a complex rearrangement of multiple atoms in concerted manner. Such a feature is strikingly different from any switches mediated by single-atom/molecule processes that have been previously reported. The ultimate goal of nanoelectronics is the miniaturization of electronic components and their integration into more complex devices. To reach this goal, scanning probe microscopies (SPM), such as scanning tunnelling microscopy (STM) and atomic force microscopy (AFM), have been used not only to characterize but also to manipulate individual atoms and molecules on a surface. To date, a number of atomic-scale manipulations have been reported, where precisely controlled SPM tip-surface interactions are utilized to move single atoms/molecules on surfaces in vertical and lateral directions. As reported in the previous studies, these interactions result in highly controllable processes, such as fabrication of artificial atomic-scale structures [1] , [2] , [3] , [4] , [5] and control of quantum phenomena [6] , [7] , [8] , [9] , demonstrating the promising capability of SPM to fabricate atomic-scale functional devices. As a fundamental functional unit, the atomic-scale switch has attracted great interest for its potential application as a logic gate or memory cell. The first prototype was reported in 1991 in an STM study [10] , where it was shown that applying voltage pulses with opposite polarity could transfer a single xenon atom back and forth between an STM tip and a nickel surface. Since this pioneering work, extensive studies using STM/AFM have demonstrated a variety of atomic-scale switches composed of not only an adsorbed atom but also adsorbed molecules and native surface atoms. In all cases, reversible switches could be operated in a controlled way through their single-atom/molecule processes such as lateral/vertical displacements [11] , [12] , [13] , [14] , rotational motions [15] , [16] , [17] and conformational changes [18] , [19] , [20] . Nevertheless, most switches devised thus far need to be operated at cryogenic temperatures, while controllability at room-temperature (RT) environment is essential for the many practical applications that await this new technology. The intractable obstacles for high-performance atomic-scale switch at RT are the uncontrollable processes predominant at increased temperatures, such as thermal switching [21] , [22] , [23] , thermal diffusion [24] , [25] , [26] and thermal dissociation [27] . Suppressing these processes still remains a challenge. Here we report an atomic-scale switch, composed of a binary Pb/Si cluster on the Si(111)-(7 × 7) surface. The binary cluster is assembled using atomic-level manipulation, and is operated as an RT switch using a tunnelling carrier injection from an SPM tip. The created switch undergoes concerted atom exchanges and displacements, which is strikingly different from any reported switches involving single-atom/molecular processes. Moreover, bidirectional and unidirectional switch motions can be regulated by selecting electron or hole injection through different inelastic reaction channels. Our approach, fabricating an electrically operable RT switch at an atomically precise position, constitutes a further step towards the development of atomic-scale integrated electronics for use at RT. Constructing an atomically size-defined Pb cluster Extensive SPM studies have reported a variety of methods for single-atom/molecule manipulation that are mediated by several tip–sample interactions [1] , [2] , [28] , [29] . We used a combined AFM/STM to fabricate and operate an atomic-scale switch at RT, which enables individual interactions during each manipulation process to be directly monitored. A metal (Pt–Ir)-coated Si cantilever was oscillated at its resonance frequency with constant amplitude, and the time-averaged tunnelling current ( I t ) and frequency shift (Δ f ) of the cantilever oscillation were simultaneously measured [30] . Bias voltage ( V s ) was applied to the sample with respect to the tip at the ground. An RT switch was created by assembling a Pb nanocluster from single Pb atoms adsorbed on an Si(111)-(7 × 7) surface. Semiconductor substrates can be utilized to suppress the thermal mobility of adsorbates because they exhibit highly corrugated potential-energy surfaces [31] . 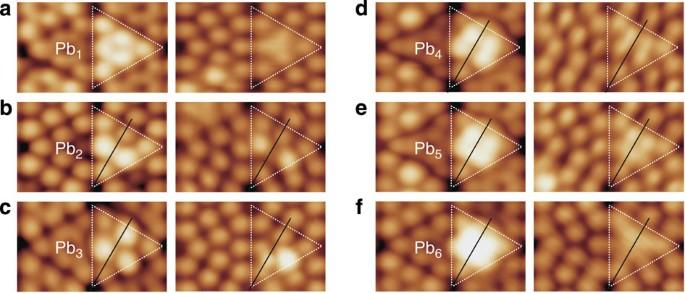Figure 1: Pb nanoclusters constructed by successive atom manipulations. (a–f) STM topographic images of typical Pb1–Pb6clusters assembled in a faulted HUC (dashed triangles) of the Si(111)-(7 × 7) surface acquired atIt=20 pA. Sample biases were set atVs=−1.0 V (left) andVs=+1.0 V (right). Image size 3.0 by 5.0 nm. Figure 1a shows (left) filled- and (right) empty-state STM images of a single Pb atom on an Si(111)-(7 × 7) surface. A single Pb atom is confined in one half-unit cell (HUC) while thermally hopping within the HUC at a much faster rate than the SPM scanning speed, resulting in a time-averaged image at RT. This is because the thermal energy of a single Pb atom at RT is smaller than the potential barrier between adjacent HUCs but larger than that between adjacent adsorption sites in the HUC [22] , [24] . Figure 1: Pb nanoclusters constructed by successive atom manipulations. ( a – f ) STM topographic images of typical Pb 1 –Pb 6 clusters assembled in a faulted HUC (dashed triangles) of the Si(111)-(7 × 7) surface acquired at I t =20 pA. Sample biases were set at V s =−1.0 V (left) and V s =+1.0 V (right). Image size 3.0 by 5.0 nm. Full size image To construct nanoclusters, we used an SPM tip to mechanically manipulate single Pb atoms [32] . Pb atoms were collected one by one into a predetermined HUC (further information can be found in Supplementary Figs 1–3 and Supplementary Note 1 and 2 ), which gave us direct insight into the exact number of constituent atoms (cluster size). Figure 1b–f summarizes (left) filled- and (right) empty-state STM images of constructed Pb n ( n =2–6) nanoclusters, where n denotes the cluster size. As described above, Pb 1 is hopping fast inside the HUC. The hopping rate can be estimated from the extrapolated value of the previous report [22] as ~6.7 × 10 6 s −1 . From Pb 2 onwards, Pb atoms practically stop hopping and show cluster-like structures. However, Pb 2 still shows thermal fluctuation at the rate of ~1.9 × 10 −4 s −1 (see Supplementary Fig. 4a and Supplementary Note 3 ). This rate, which agrees well with that found in a previous report (~3.1 × 10 −4 s −1 ) [21] , is 10 orders smaller than the Pb 1 -hopping rate. Thus, Pb 2 is thermally unstable at RT, although dimerization drastically suppresses the fluctuation. While Pb 3 was stably imaged at small | V s |, the conformation changed when imaged at V s =1.0 V (see Supplementary Fig. 4b,c and Supplementary Note 3 ). Thus, Pb 3 is at least thermally stable at RT, but is still reactive to the tip current (described in detail later). On the other hand, Pb n ( n =4,5,6) were imaged without any changes irrespective of V s (−2.0 V≤ V s ≤2.0 V), and thus can be considered stable against both thermal fluctuation and tip perturbations. These results clearly show that Pb nanoclusters tend to be stable with increasing numbers of constituent Pb atoms, showing a strong size effect. Atomic structure of Pb trimer To operate an atomic-scale switch at RT, stability against thermal fluctuation and reactivity by tip perturbations are essential. In this sense, Pb 3 is eligible for application as an RT switch. For a filled-state image, Pb 3 appears as three bright spots at centre adatom (Ce) sites. In contrast, the empty state has a different appearance characterized by a larger spot at one Ce site and a smaller spot near one rest atom site. It is evident that the Pb 3 loses the mirror symmetry preserved in other size clusters [Pb n ( n =2,4,5,6)]; that is, the Pb nanocluster exhibits a chiral channel only by trimerization. We performed density functional theory calculations to determine the structure of Pb 3 on the Si(111)-(7 × 7) surface. Preferential adsorption sites of single Pb atoms are known as high-coordination sites around rest atoms [22] . Although we first adapted these sites to calculate possible Pb 3 structures, none of them reproduced the drastic contrast change observed between filled- and empty-state images (see Supplementary Fig. 5 and Supplementary Note 4 ). This prompted us to reconsider the structure including Pb substitutions, since a single Pb atom will replace a substrate Si adatom at a few 100 ° C, and the contrast pattern strongly depends on V s (see Supplementary Fig. 7 and Supplementary Note 5 ). Among the several models considered (see Supplementary Fig. 5 ), only one nicely reproduced the observed filled- and empty-state STM images ( Fig. 2a,b ). The corresponding model ( Fig. 2c ) reveals that trimerization promotes Pb–Si exchanges at two Ce sites. Thus, the Pb 3 is no longer a single-element cluster but a binary cluster composed of Pb and Si atoms. 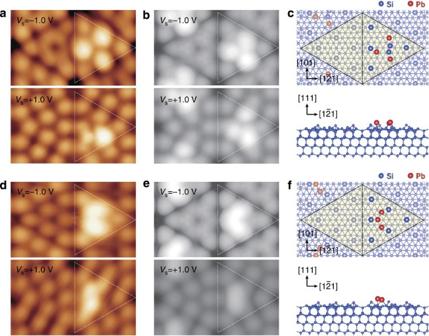Figure 2: Atomic structures of Pb trimers. (a) Topographic STM images (It=20 pA) of a Pb3confined in a faulted HUC (dashed triangles) acquired atVs=−1.0 V (top) and +1.0 V (bottom), respectively. (b) Calculated STM topographic images using structural model incatVs=−1.0 V (top) and +1.0 V (bottom), respectively. (c) Top view (top) and side view (bottom) of the proposed atomic structure of the Pb3cluster on an Si(111)-(7 × 7) surface. (d) Topographic STM images (It=20 pA) of a metastable Pb trimer confined in a faulted HUC (dashed triangles) acquired atVs=−1.0 V (top) and +1.0 V (bottom), respectively. (e) STM topographic images calculated using the structural model infatVs=−1.0 V (top) and +1.0 V (bottom), respectively. (f) Top view (top) and side view (bottom) of the proposed atomic structure of the cluster on the Si(111)-(7 × 7) surface. Figure 2: Atomic structures of Pb trimers. ( a ) Topographic STM images ( I t =20 pA) of a Pb 3 confined in a faulted HUC (dashed triangles) acquired at V s =−1.0 V (top) and +1.0 V (bottom), respectively. ( b ) Calculated STM topographic images using structural model in c at V s =−1.0 V (top) and +1.0 V (bottom), respectively. ( c ) Top view (top) and side view (bottom) of the proposed atomic structure of the Pb 3 cluster on an Si(111)-(7 × 7) surface. ( d ) Topographic STM images ( I t =20 pA) of a metastable Pb trimer confined in a faulted HUC (dashed triangles) acquired at V s =−1.0 V (top) and +1.0 V (bottom), respectively. ( e ) STM topographic images calculated using the structural model in f at V s =−1.0 V (top) and +1.0 V (bottom), respectively. ( f ) Top view (top) and side view (bottom) of the proposed atomic structure of the cluster on the Si(111)-(7 × 7) surface. Full size image We have also confirmed that Pb 3 is stabilized by being a binary cluster. Figure 2d shows (top) filled- and (bottom) empty-state STM images of a Pb trimer just after construction, which exhibit different appearances from those of Pb 3 in Fig. 2a . This Pb trimer, denoted by Pb 3 *, fluctuates in its conformation, and lasts only a few tens of minutes, followed by transition to Pb 3 (see Supplementary Fig. 8 and Supplementary Note 6 ). Figure 2e shows the calculated (top) filled- and (bottom) empty-state STM images, which well reproduce the observed Pb 3 * appearances. The corresponding model ( Fig. 2f ) reveals that the structure contains no substitutional Pb atoms, and thus is regarded as a single-element cluster. These results clearly indicate that the Pb 3 * is in a metastable state before stabilization to the Pb 3 via Pb–Si exchanges. Current induced switch of the Pb trimer Owing to the symmetry of the 7 × 7 structure, Pb 3 exists as six conformations (see Supplementary Fig. 9 and Supplementary Note 7 ). We revealed that the Pb 3 conformation switches reversibly between particular pairs by imaging at V s exceeding apparent thresholds. The switch pair is shown in Fig. 3a,b , which we denote as L and R , respectively. The switch was triggered when the tip was scanned over the substitutional Pb (Pb sub ) site (red cross in Fig. 3a,b ) or substitutional Si (Si sub ) site (blue cross in Fig. 3a,b ). Since the L and R states are nonsuperimposable mirror images of one another by translation and rotation, the present switch is an inversion between opposite chiral states (chiral switch). It is also noteworthy that the chiral inversion is not a simple rotation or displacement of the whole Pb 3 configuration but rather a complex motion involving two Pb and three Si atoms, where Pb–Si exchanges and Pb- and Si displacements are indeed promoted in concert. This feature is strikingly different from any reported switches involving only single-atom/molecule processes [10] , [11] , [12] , [13] , [14] , [15] , [16] , [17] , [18] , [19] , [20] , thus being a new type of switch. 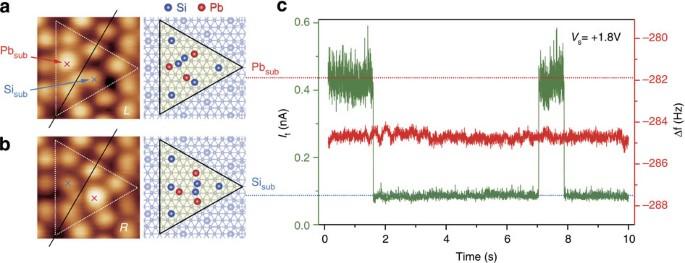Figure 3: Concerted switch of Pb3. (a,b; Left) Experimental STM topographic images (It=20 pA andVs=+0.5 V) and (right) the corresponding structural models derived from the density functional theory calculation, showing a pair of conformational switching. The two conformations are distinguished by the labelsL(a) andR(b). Solid lines in STM images indicate the chiral axes. Red and blue crosses show the substitutional Pb (Pbsub) site and the substitutional Si (Sisub) site, respectively. (c) Simultaneous current and frequency-shift traces (switch time chart) during the voltage pulse application (Vs=+1.8 V). Through the measurement, the tip was fixed at identical sites (the Pbsubsite in theLstate and the Sisubsite in theRstate). The high- and low-current states correspond to theL(a) andR(b) states, respectively. Figure 3: Concerted switch of Pb 3 . ( a , b ; Left) Experimental STM topographic images ( I t =20 pA and V s =+0.5 V) and (right) the corresponding structural models derived from the density functional theory calculation, showing a pair of conformational switching. The two conformations are distinguished by the labels L ( a ) and R ( b ). Solid lines in STM images indicate the chiral axes. Red and blue crosses show the substitutional Pb (Pb sub ) site and the substitutional Si (Si sub ) site, respectively. ( c ) Simultaneous current and frequency-shift traces (switch time chart) during the voltage pulse application ( V s =+1.8 V). Through the measurement, the tip was fixed at identical sites (the Pb sub site in the L state and the Si sub site in the R state). The high- and low-current states correspond to the L ( a ) and R ( b ) states, respectively. Full size image To explore the switch reaction, we carried out the following measurement. First, the initial conformation was imaged at V s =0.5 V. Then, the tip was fixed at a selected site, and a square voltage pulse (−1.8 V≤ V s ≤2.0 V) of typically 10-s duration was applied to the surface with the z-feedback loop opened. During the voltage pulse, I t and Δ f were recorded simultaneously. After the measurement, rescanning the same area at V s =0.5 V revealed the resulting conformation. The switch time chart at V s =1.8 V is presented in Fig. 3c , where the tip was initially fixed at the Pb sub site in the L state. Through the measurement, I t switches between high and low levels, which correspond to the L ( Fig. 3a ) and the R ( Fig. 3b ) states, respectively. Interestingly, such bidirectional switches alternatively change the atom below the fixed tip between Pb sub (red cross in Fig. 3a ) and Si sub (blue cross in Fig. 3b ). 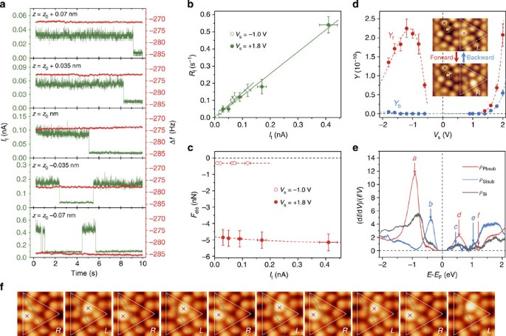Figure 4: Characteristics of the Pb3switch. (a) Tip–sample distance dependences of the current (green) and frequency-shift (red) traces during the voltage pulse of +1.8 V.z0indicates the feedback tip–sample distance atIt=20 pA andVs=+0.5 V. (b) Current dependences of the forward-switch rate atVs=+1.8 V (solid circle) andVs=−1.0 V (open circle). Solid lines are linear fits of the data. Vertical error bars represent the s.e.m. for the measurements repeated up to 20 times per data point, and horizontal ones, s.e.m. for the measured current in theLstate. (c) Current dependences of the tip–sample electrostatic force atVs=+1.8 V (solid circle) andVs=−1.0 V (open circle). Dashed lines are guides to the eye. Vertical error bars are s.e.m. derived from the systematic uncertainty in the measurements of the cantilever oscillation amplitude and cantilever stiffness. Horizontal error bars are identical with those inb. (d) Yields of the forward (red circle) and backward (blue circle) switches as a function of pulse bias voltage. Red and blue dashed lines are guides to the eye. Red (blue) cross in the STM images shows an active site for forward (backward) switch. Black cross indicates a centre Si adatom site without Pb occupation. Error bars were estimated by an error-propagation analysis from the errors in theRf(b)andIt. (e) Local density of states acquired at red (ρPbsub), blue (ρSisub) and black (ρSi) crossed sites ind. Fermi level (EF) is referenced to energy zero. Typical peaks or onsets of the spectra are labelleda–f. (f) STM topographies of a Pb3(It=40 pA andVs=+0.5 V) imaged at the intervals of 10-s voltage pulse applications (Vs=−1.4 V). Red cross in each image indicates a fixed tip position during the voltage pulse. Solid line in each image indicates a chiral axis. Figure 4a shows the switch time charts acquired at different tip–sample separations ( z ). With the tip approaching the surface (from top to bottom), I t increases and the switch occurs more frequently. From such current traces, we analysed the rate of forward ( L → R ) and backward ( R → L ) switching by a simple form as R f(b) = N f(b) / τ L(R) , where N f(b) is the total number of forward (backward) switches and τ L(R) is the total residence time in the L ( R ) state. R f as a function of I t is shown in Fig. 4b . For both bias polarities, the switch rates on the current are linear, suggesting a single-carrier (electron or hole) process driving the switch. Figure 4: Characteristics of the Pb 3 switch. ( a ) Tip–sample distance dependences of the current (green) and frequency-shift (red) traces during the voltage pulse of +1.8 V. z 0 indicates the feedback tip–sample distance at I t =20 pA and V s =+0.5 V. ( b ) Current dependences of the forward-switch rate at V s =+1.8 V (solid circle) and V s =−1.0 V (open circle). Solid lines are linear fits of the data. Vertical error bars represent the s.e.m. for the measurements repeated up to 20 times per data point, and horizontal ones, s.e.m. for the measured current in the L state. ( c ) Current dependences of the tip–sample electrostatic force at V s =+1.8 V (solid circle) and V s =−1.0 V (open circle). Dashed lines are guides to the eye. Vertical error bars are s.e.m. derived from the systematic uncertainty in the measurements of the cantilever oscillation amplitude and cantilever stiffness. Horizontal error bars are identical with those in b . ( d ) Yields of the forward (red circle) and backward (blue circle) switches as a function of pulse bias voltage. Red and blue dashed lines are guides to the eye. Red (blue) cross in the STM images shows an active site for forward (backward) switch. Black cross indicates a centre Si adatom site without Pb occupation. Error bars were estimated by an error-propagation analysis from the errors in the R f(b) and I t . ( e ) Local density of states acquired at red ( ρ Pbsub ), blue ( ρ Sisub ) and black ( ρ Si ) crossed sites in d . Fermi level ( E F ) is referenced to energy zero. Typical peaks or onsets of the spectra are labelled a – f . ( f ) STM topographies of a Pb 3 ( I t =40 pA and V s =+0.5 V) imaged at the intervals of 10-s voltage pulse applications ( V s =−1.4 V). Red cross in each image indicates a fixed tip position during the voltage pulse. Solid line in each image indicates a chiral axis. Full size image AFM/STM allows us to directly examine other possible tip effects in the present switch, such as short-range force ( F SR ), van der Waals force ( F vdW ) and electrostatic force ( F ele ). Among them, F SR and F vdW depend on z but are independent of V s . Since the present switch occurred only by applying higher voltage, while z was fixed, the effects of these mechanical interactions are easily excluded. In Fig. 4a , Δ f , which remains unchanged but slightly alters with z , is caused mainly by F ele and F vdW . To examine the possible role of electrostatic force, F ele in such Δ f signals was extracted on the basis of the force decomposition method [33] (see Supplementary Fig. 10 and Supplementary Note 8 ). Figure 4c shows F ele as a function of I t during the voltage pulse. For both polarities, | F ele | increases with I t , but the change is negligibly small over the whole I t range, whereas the switch rates increase clearly ( Fig. 4b ). The enhancement rate of F ele was only 6% (5%) with increasing I t from 0.03(0.01) to 0.41(0.12) nA at V s =1.8 V (−1.0 V). The result definitely rules out the electric field-induced effect, confirming that the switch is driven exclusively by carrier injection from the tip to the surface. To characterize the switch behaviour, the quantum yields of forward (backward) switch [ Y f(b) = eR f(b) / I t ] were investigated at different V s values ( Fig. 4d ). For positive V s , both Y f (red circles) and Y b (blue circles) increase exponentially above an apparent threshold bias ( V s =1.0 V) up to V s =2.0 V. Thus, electrons induce a bidirectional switch. For negative V s , by contrast, Y f forms a peak around V s =−1.2 V, while Y b remains almost zero and only slightly increases below V s =−1.5 V. Thus, hole injection induces the switch only at the Pb sub site but not at the Si sub site, resulting in a unidirectional switch behaviour. This feature enabled us to control the chiral states as shown in Fig. 4f where the image array from the left to the right indicates changes in the chiral states of the same Pb 3 . Under the hole-injection condition ( V s =−1.4 V ), we successfully performed at least 30 consecutive unidirectional switches to direct L and R states alternatively. To gain insight into the mechanism of the carrier-selective switch behaviour, we measured (d I /d V )/( I / V ) spectra ( Fig. 4e ), which are proportional to the local density of states [34] . The spectrum-labelled ρ Pbsub ( ρ Sisub ) is acquired at the Pb sub (Si sub ) site, indicated by the red (blue) cross in Fig. 4d . For comparison, Fig. 4e also cites the spectrum, ρ Si , at the pristine Ce site (black cross in Fig. 4d ). Above the Fermi level, ρ Pbsub and ρ Sisub show a slight difference but the overall trends are same. The energy onsets (labelled e ( f )) roughly correspond to the threshold of Y f(b) ( Fig. 4d ), indicating that the electron injection to these electronic states results in a bidirectional switch. Below the Fermi level, in contrast, ρ Pbsub forms a remarkable peak around −1.0 eV (labelled a ), while ρ Sisub forms a peak only at lower energy, −0.3 eV (labelled b ), and slightly increases but is less pronounced below −0.7 eV. Because the switch behaviour for the hole injection is observed at the Pb sub site only, we suggest that the unidirectional switch is induced by the hole injection into Pb sub -derived states. We calculated the density of states projected on the atomic orbitals for Pb sub and Si sub . The result (see Supplementary Fig. 6 ) revealed that the peak corresponding to a in Fig. 4e is a Pb-derived resonance state (bonding state between the Pb orbital and substrate wave function) localized in the vicinity of Pb sub , while that for f ( e ) in Fig. 4e is the antibonding state for Pb sub (Si sub ) and the substrate. Our results suggest that the switch is caused by the formation of an excited electronic state by the inelastic scattering of a single electron/hole, which strongly couples to the atomic motions, a mechanism similar to desorption induced by electronic transitions [12] , [35] , [36] . Understanding of the detailed mechanism, however, requires elucidation of the complicated reaction pathway of the concerted process, and is deserved for a future work. As to the concerted switch behaviour, its occurrence is also supported by Fig. 4d . Since the energy per Pb–Si covalent bond is 0.88 eV (ref. 37 ), the onset bias, ~−0.5 V, for the present switch involving at least two Pb/Si exchanges is energetically unfavourable through a simple bond-breaking mechanism. That means reduction of the switch barrier is achieved through concerted atom motions [38] , [39] . Further, the present switch yield, ~10 −10 , is a few orders smaller than those involving single-atom/molecule processes, 10 −9 –10 −5 (refs 11 , 12 , 14 , 15 , 16 , 17 , 18 ). This is because the concerted switch yield is determined by the probability of occurrence of the complex processes [40] . Since the structural/electrical property of the system and the bias range required for the reaction also affect the yields, the relation is not explicit. Nevertheless, the decreasing yield is outstanding, which is plausible because of the concerted process. Basically, the concerted process requires the local presence of a sufficient number of reactants [39] , which is satisfied in our case by the confinement of the nanocluster and its size-dependent property. In our experiment, HUC, which serves as a 2D nanospace, discourages fragmentation of cluster-constituent atoms into individual atoms. When the cluster size becomes larger, the increasing site occupancy of the atoms interrupts the paths of the individual atom hops, and the atom–atom proximity enhances their mutual attractive interactions. Accordingly, the individual atom motions influence each other, and only their collective motion contributes to the cluster conformational change, which is the prime reason for the size-dependent cluster stability found in the present study. We suggest that the size of Pb 3 is just enough to be stabilized at RT, where the attractive interactions of the internal atoms are not so strong that the conformation becomes rigid. Therefore, additional energy input from the tunnelling carrier can trigger the internal atom motions in concert, resulting in the switching. Note that the proper adjustment of cluster size by atom-by-atom assembly is technically important to achieve such a subtle energy balance. Concerted process is fundamentally important in several microscopic phenomena on surface or in bulk, such as atom/cluster/molecule diffusion [38] and crystal/thin-film growth [39] , which are predicted to occur by the surrounding atom motions as kinetically hindered processes. Our direct observation and even control of concerted switching provide further insight into these phenomena that enhance our ability to control the surface morphology. On the other hand, our approach has a great advantage: namely, well-characterized chiral motifs constructed at atomically precise positions at RT. The method is potentially utilized to form the desired chiral templates, for example, creation of a homochiral domain/cluster and allocation of chiral motifs near some reactive elements, a pioneering new RT strategy to investigate the enantioselective interactions and reactions from a microscopic view. From a technological perspective, prominent features of the present Pb 3 switch are the high stability and the controllability at RT, that is, Pb 3 potentially works as an elementary unit of a reliable memory storage. To perform such an actual memory device, atomic-scale integration of the Pb 3 units is the most important and challenging task. We suggest that one of the promising approaches to overcome the problem is the self-assembling method [41] . This method potentially achieves the formation of a periodically well-ordered Pb 3 array on the Si(111)-(7 × 7) surface, realizing the memory device with ultra-high-density recording and reading of information at RT. Furthermore, the present method to construct a size-defined cluster is widely applicable to various elements on several surfaces. Nanoclusters are known to exhibit unique physical and chemical properties that depend strongly on their size and constituent atoms [42] , [43] , [44] , [45] , [46] . This motivates us to create a variety of atomic-scale devices with different functionalities and to systematically embed them into desired nanoregions, which opens up novel nanofabrication to achieve atomic-scale integrated electronics for RT operation. Experimental set-up All experiments were carried out using a custom-built ultrahigh-vacuum (~5 × 10 −11 torr) AFM/STM system operated at RT. The tip apex of Pt–Ir-coated Si cantilever (NCLPt, NanoWorld) was carefully cleaned by Ar ion sputtering before use. The cantilever deflection sensor is on the basis of an optical interferometer. For AFM/STM measurements, we applied a frequency modulation detection method that simultaneously records the Δ f of cantilevers oscillating at a constant amplitude and the average of the time-varying current I t between the tip and the sample. The thermal drift during data acquisition was compensated by a combination of atom-tracking and feed-forward techniques [47] , using a home-built software programme. The clean Si(111)-(7 × 7) surface (Sb-doped, resistivity <0.02 Ωcm) was prepared by the standard method of degassing followed by flash annealing. Pb atoms (~3 × 10 −4 ML) were deposited at RT by a Joule heating evaporator. The pressure was kept under 10 −10 torr during evaporation. Theoretical calculations All the density functional theory calculations were performed using the STATE code [48] . The Perdew–Burke–Ernzerhof [49] exchange correlation functional was used. STM simulations were based on the Tersoff–Hamann theory [50] . A detailed description of the theoretical calculations can be found in the Supplementary Note 4 . How to cite this article: Inami, E. et al . Room-temperature-concerted switch made of a binary atom cluster. Nat. Commun. 6:6231 doi: 10.1038/ncomms7231 (2015).